Escherichia colinoncoding RNAs can affect gene expression and physiology ofCaenorhabditis elegans Food and other environmental factors affect gene expression and behaviour of animals. Differences in bacterial food affect the behaviour and longevity of Caenorhabditis elegans . However, no research has been carried out to investigate whether bacteria could utilize endogenous RNAs to affect C. elegans physiology. Here we show that two Escherichia coli endogenous noncoding RNAs, OxyS and DsrA, impact on the physiology of C. elegans . OxyS downregulates che-2 , leading to impairment in C. elegans chemosensory behaviour and DsrA suppresses diacylglycerol lipase gene F42G9.6 , leading to a decrease in longevity. We also examine some genes in the C. elegans RNA interference pathway for their possible involvement in the effects of OxyS and DsrA. Other bacteria, such as Bacillus mycoides , may also utilize its noncoding RNAs to interfere with gene expression in C. elegans . Our results demonstrate that E. coli noncoding RNAs can regulate gene expression and physiological conditions of C. elegans and indicate that noncoding RNAs might have interspecies ecological roles. Understanding interactions between animals and their environmental factors is a central theme of biological research. Food is one of the crucial environmental factors and can affect gene expression and physiology of animals [1] , [2] . For example, high-fat diet in male rats can affect the β-cell functions of their female offspring [1] . The growth condition of Escherichia coli , a food of Caenorhabditis elegans , could interfere with sex determination of C. elegans [2] . In most cases, we still know little about the identity of the exact environmental trigger and the molecular mechanism behind these phenomena. C. elegans and some other organisms are sensitive to environmental RNA interference (RNAi) [3] . Environmental RNAi, in principle, is a physiological reaction of a species to the double-stranded RNA (dsRNA) in its environment. For C. elegans , RNAi could be achieved by soaking animals in a dsRNA solution, or by feeding them with recombinant E. coli -expressing dsRNA [4] , [5] . Some small regulatory RNAs, induced in bacteria (for example, E. coli ) under stress conditions such as oxidative stress and low temperature, activate or repress the expression of multiple genes to protect bacteria from harsh environments [6] , [7] . We speculated that these noncoding RNAs (ncRNAs) in bacteria might interfere with the physiology of bacterial foragers such as C. elegans and might serve as innate-protective factors, considering that artificially engineered dsRNAs can enter into C. elegans and suppress the expression of worm genes through a mechanism of feeding RNAi [5] . Here, we report that two E. coli endogenous ncRNAs, OxyS and DsrA, altered the physiological functions of C. elegans via regulating gene expression of the nematode. OxyS impaired C. elegans chemosensory by suppressing the expression of chemosensory gene che-2 . DsrA decreased C. elegans longevity by suppressing the expression of diacylglycerol lipase gene F42G9.6 . Both ncRNAs are expressed in E. coli under stress conditions, and may protect E. coli from overfeeding by C. elegans . OxyS-expressing E. coli alters C. elegans behaviour E. coli under oxidative stress expresses a ncRNA, OxyS, to modulate gene expression and protect cells from oxidative damage [6] , [8] . We set up behavioural assays with four E. coli strains: K12 ( wild-type ), OxyR (produce OxyS constitutively without oxidative stress), OxyS (overexpress OxyS without oxidative stress with an OxyS plasmid) and ΔOxyS (OxyS deletion strain). Wild-type N2 worms could find K12, OxyR, OxyS or ΔOxyS bacteria in a similar period of time in food quality assays, indicating that C. elegans could generally 'accept' these four strains as food sources ( Fig. 1a ). We then assessed the preference of C. elegans when they were given a choice between K12 and one of the other three strains ( Fig. 1b ). N2 worms gradually avoided staying on OxyR and OxyS strains, but did not discriminate between K12 and ΔOxyS strains ( Fig. 1b ). The degree of repulsion over the time period was correlated with the expression levels of OxyS, as OxyS strain expressing higher levels of OxyS than OxyR strain [8] repelled C. elegans more strongly ( Fig. 1b ). 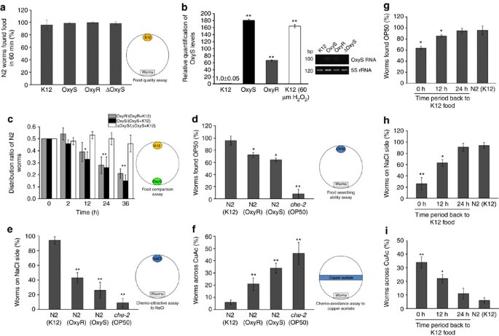Figure 1: OxyS-expressingE. colihas a physiological impact onC. elegans. (a) The fourE. colistrains could be found by N2 worms equally well as food sources.N=40 worms for each group. Setup for the 'food quality assay' (using K12 as an example for theE. colistrain tested) is shown in the right panel. (b) Real-time PCR (left) and semi-quantitative reverse transcriptase–PCR (right) revealed OxyS expression levels of K12, OxyS, OxyR, ΔOxyS and K12E. colitreated with 60 μM H2O2. (c) N2 worms were repelled from OxyS-expressingE. coli(OxyR and OxySE. coli) in the food comparison assays, whereas OxyS deletion mutantE. coli(ΔOxyS) showed no effect.N=36 worms for each group. Setup for the 'food comparison assay' (using OxyS and K12 as examples for the two strains compared) is shown in the right panel. (d) N2 worms fed with OxyS-expressingE. colishowed decreased ability in finding OP50 food. Setup for the 'food searching assay' is shown in the right panel.N=50 worms for each group. (e) N2 worms fed with OxyS-expressingE. colishowed decreased chemotaxis to NaCl. Setup for the 'chemo-attractive assay' with NaCl gradient is shown in the right panel. (f) N2 worms fed with OxyS-expressingE. colishowed decreased chemo-avoidance to copper acetate. Setup for the 'chemo-avoidance assay' with copper acetate barrier is shown in the right panel.N=30 worms ine,f. N2 worms fed continuously (48 h) with the respectiveE. colistrain were used, and data fromche-2worms fed with OP50 were also shown ind–f. (g–i) Chemosensory ability impaired by OxyS could be restored gradually when food with OxyS expression was replaced by food without OxyS expression (K12) examined with food searching assays (g), chemo-attractive assay with NaCl gradient (h) and chemo-avoidance assay with copper acetate barrier (i).N=40 worms forg–i. L4 worms were used for all behavioural assays.Pvalues were determined with two-tailed Student'st-test. *P<0.05; **P<0.01. All data are from three repeats. Error bars represent s.e.m. Figure 1: OxyS-expressing E. coli has a physiological impact on C. elegans . ( a ) The four E. coli strains could be found by N2 worms equally well as food sources. N =40 worms for each group. Setup for the 'food quality assay' (using K12 as an example for the E. coli strain tested) is shown in the right panel. ( b ) Real-time PCR (left) and semi-quantitative reverse transcriptase–PCR (right) revealed OxyS expression levels of K12, OxyS, OxyR, ΔOxyS and K12 E. coli treated with 60 μM H 2 O 2 . ( c ) N2 worms were repelled from OxyS-expressing E. coli (OxyR and OxyS E. coli ) in the food comparison assays, whereas OxyS deletion mutant E. coli (ΔOxyS) showed no effect. N =36 worms for each group. Setup for the 'food comparison assay' (using OxyS and K12 as examples for the two strains compared) is shown in the right panel. ( d ) N2 worms fed with OxyS-expressing E. coli showed decreased ability in finding OP50 food. Setup for the 'food searching assay' is shown in the right panel. N =50 worms for each group. ( e ) N2 worms fed with OxyS-expressing E. coli showed decreased chemotaxis to NaCl. Setup for the 'chemo-attractive assay' with NaCl gradient is shown in the right panel. ( f ) N2 worms fed with OxyS-expressing E. coli showed decreased chemo-avoidance to copper acetate. Setup for the 'chemo-avoidance assay' with copper acetate barrier is shown in the right panel. N =30 worms in e , f . N2 worms fed continuously (48 h) with the respective E. coli strain were used, and data from che-2 worms fed with OP50 were also shown in d – f . ( g – i ) Chemosensory ability impaired by OxyS could be restored gradually when food with OxyS expression was replaced by food without OxyS expression (K12) examined with food searching assays ( g ), chemo-attractive assay with NaCl gradient ( h ) and chemo-avoidance assay with copper acetate barrier ( i ). N =40 worms for g – i . L4 worms were used for all behavioural assays. P values were determined with two-tailed Student's t -test. * P <0.05; ** P <0.01. All data are from three repeats. Error bars represent s.e.m. Full size image The repulsion to C. elegans by OxyS-expressing E. coli might result from suppression of food searching ability in C. elegans , that is, worms with impaired food searching ability might be easier to gradually wander off from OxyS-expressing bacteria, and eventually end up accumulating on bacteria without OxyS expression. We therefore examined the effect of continuous feeding of OxyS or OxyR E. coli to C. elegans . N2 worms fed for 2 days on OxyS-expressing bacteria had an impaired ability to find OP50 in food searching ability assays ( Fig. 1d ). Food searching is generally associated with locomotion and chemosensory in C. elegans [9] . Chemosensory assays showed that N2 worms fed with OxyS-expressing strains exhibited defects in chemo-attraction to NaCl and chemo-avoidance to copper acetate ( Fig. 1e ). Chemosensory ability impaired by OxyS RNA could be gradually restored when food with OxyS expression was replaced by that without OxyS expression ( Fig. 1g–i ). Thus, in the food comparison assays, once on the food without OxyS expression, worms would gradually recover from the impairment on chemosensory and tend to remain on this food. No defect was observed in locomotion of N2 worms fed with OxyS-expressing E. coli in locomotion assays (data not shown). These results suggest that C. elegans fed on OxyS-expressing E. coli had impaired chemosensory ability. OxyS downregulates C. elegans chemosensory gene che-2 We searched known E. coli small regulatory RNA sequences against the C. elegans transcripts ( Supplementary Table S1 ). che-2 was identified as the only mRNA harbouring a continuous 17-nucleotide (nt) sequence complementary to OxyS in blast sequence analysis ( Fig. 2a ). che-2 encodes a member of the WD40 protein family, and affects chemosensory in C. elegans , with che-2(e1033) worms showing significant defects in chemosensory abilities [10] . In food searching ability assays, around 10–20% che-2(e1033) worms could find OP50 food within 90 min, in contrast to nearly 100% for N2 worms ( Fig. 1d ). che-2(e1033) were also deficient in chemo-attractance to NaCl and chemo-avoidance to copper acetate ( Fig. 1e ). We fed a Pche-2::che-2::gfp transgenic line with K12, OxyR or OxyS E. coli , and found that there was a decreased intensity of green fluorescent protein (GFP) signal in worms fed with OxyR or OxyS strain compared with K12 ( Fig. 2c ). Western blots confirmed this reduction ( Fig. 2d ). Furthermore, decline of che-2 mRNA was detected in N2 worms fed with OxyS-expressing E. coli ( Fig. 2e ). As che-2 downregulation may result from a decrease in transcription or che-2 mRNA degradation, transgenic animals with the che-2 promoter fused to a GFP reporter ( Pche-2::gfp ) were constructed to distinguish these two possibilities. There was no reduction of GFP signal observed in Pche-2::gfp transgenic lines fed with OxyR or OxyS bacteria compared with K12 feeding (data not shown); thus, che-2 transcription may not be affected. We also examined the expression of sym-1 and cdh-12 by real-time PCR. These two genes are among several other genes that have comparable stretches of identity to OxyS, but do not harbour a continuous 17-nt or longer complementary sequence to OxyS like che-2 . No significant difference in their expression levels was found between worms fed on E. coli with or without OxyS expressing ( Supplementary Fig. S1 ). 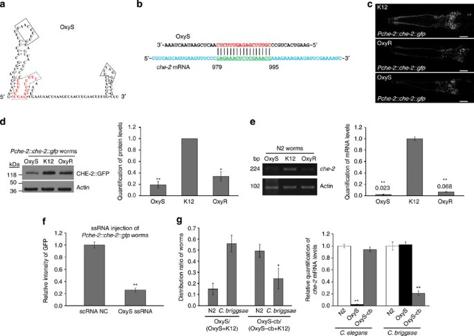Figure 2: OxyS RNA suppresses the expression ofche-2. (a) Structure of OxyS. Boxed sequences are functional sites for targeting mRNAs inE. coli; sequence in dotted box is complementary toche-2mRNA. (b) Complementary sequence between OxyS andche-2mRNA; nucleotides onche-2mRNA are numbered from the start codon as +1. (c) Representative GFP images to show that GFP expression decreased inPche-2::che-2::gfpworms fed with OxyR and OxySE. coli. Animals were photographed 36 h after continuous feeding. GFP images were taken with same parameters. Scale bar is 50 μm. (d) Western blot shows decreased CHE-2::GFP protein levels inPche-2::che-2::gfpworms fed with OxyR and OxyS (left), quantification of the western blots from three repeats was also shown (right) and values form K12-fed animals were normalized to 1.0. (e) Semi-quantitative reverse transcriptase–PCR (left) and real-time PCR (right) decreasedche-2mRNA levels in N2 worms fed with OxyR and OxySE. coli.che-2mRNA level (normalized with actin) from K12-fed animals is defined as 1.0. (f) Relative quantification of GFP intensity shows that injection of the OxyS RNA decreased GFP expression inPche-2::che-2::gfpworms. A modified OxyS containing a scrambled sequence in the region predicted to targetche-2was used as a negative control (OxyS-NC). GFP images were taken with the same parameters.N=20 worms for each group. (g) OxySE. colirepelledC. elegansbut notC. briggsae, whereas OxyS-cb-expressingE. colirepelledC. briggsaebut notC. elegansin food comparison assays (left panel).N=36 worms. Right panel, real-time PCR ofC. elegansandC. briggsae che-2mRNA. OxyS-expressingE. colidecreasedC. elegans che-2mRNA level, whereas OxyS-cb suppressedC. briggsae che-2.Pvalues were determined by two-tailed Student'st-test. *P<0.05; **P<0.01. All data are from three repeats. Error bars represent s.e.m. Figure 2: OxyS RNA suppresses the expression of che-2 . ( a ) Structure of OxyS. Boxed sequences are functional sites for targeting mRNAs in E. coli ; sequence in dotted box is complementary to che-2 mRNA. ( b ) Complementary sequence between OxyS and che-2 mRNA; nucleotides on che-2 mRNA are numbered from the start codon as +1. ( c ) Representative GFP images to show that GFP expression decreased in Pche-2::che-2::gfp worms fed with OxyR and OxyS E. coli . Animals were photographed 36 h after continuous feeding. GFP images were taken with same parameters. Scale bar is 50 μm. ( d ) Western blot shows decreased CHE-2::GFP protein levels in Pche-2::che-2::gfp worms fed with OxyR and OxyS (left), quantification of the western blots from three repeats was also shown (right) and values form K12-fed animals were normalized to 1.0. ( e ) Semi-quantitative reverse transcriptase–PCR (left) and real-time PCR (right) decreased che-2 mRNA levels in N2 worms fed with OxyR and OxyS E. coli . che-2 mRNA level (normalized with actin) from K12-fed animals is defined as 1.0. ( f ) Relative quantification of GFP intensity shows that injection of the OxyS RNA decreased GFP expression in Pche-2::che-2::gfp worms. A modified OxyS containing a scrambled sequence in the region predicted to target che-2 was used as a negative control (OxyS-NC). GFP images were taken with the same parameters. N =20 worms for each group. ( g ) OxyS E. coli repelled C. elegans but not C. briggsae , whereas OxyS-cb-expressing E. coli repelled C. briggsae but not C. elegans in food comparison assays (left panel). N =36 worms. Right panel, real-time PCR of C. elegans and C. briggsae che-2 mRNA. OxyS-expressing E. coli decreased C. elegans che-2 mRNA level, whereas OxyS-cb suppressed C. briggsae che-2 . P values were determined by two-tailed Student's t -test. * P <0.05; ** P <0.01. All data are from three repeats. Error bars represent s.e.m. Full size image Worms did not show discrimination to boiled or ultrviolet (UV)-killed bacteria no matter whether they expressed OxyS or not. We added in vitro synthesized OxyS RNA to one dead bacteria spot, and added the other dead bacteria spot with a negative control RNA in the food comparison assays, and worms showed avoidance to OxyS-coated dead bacteria ( Supplementary Fig. S2 ). Real-time PCR also revealed a decrease in che-2 mRNA levels in worms fed with OxyS-coated dead bacteria ( Supplementary Fig. S2 ). In addition, injection of OxyS synthesized in vitro into the Pche-2::che-2::gfp transgenic line reduced the GFP signal ( Fig. 2f ), indicating that OxyS alone was sufficient to inhibit che-2 expression. Taken together, we conclude that OxyS inhibits C. elegans chemosensory through che-2 suppression by affecting the mRNA level probably through promoting mRNA degradation, although inhibition at the transcriptional level requiring the genomic coding region or nascent transcript could not be ruled out. The che-2 homologue in Caenorhabditis briggsae does not harbour the complete OxyS complementary site, and C. briggsae exhibited no preference between K12- and OxyS-expressing E. coli ( Fig. 2g ). Interestingly, when the 17-nt sequence complementary to the C. elegans che-2 in OxyS was changed to complement the C. briggsae che-2 (OxyS-cb) sequence ( Supplementary Fig. S1 ), OxyS-cb-expressing E. coli repelled C. briggsae moderately ( Fig. 2g ). Consistent with data from the behavioural assays, OxyS-cb-expressing E. coli lowered che-2 mRNA levels in C. briggsae , but not in C. elegans ( Fig. 2g ). Dead E. coli conditioned with in vitro synthesized OxyS-cb or OxyS (as a negative control) was used to test C. briggsae , and OxyS-cb showed 'repulsion' in the food comparison assays ( Supplementary Fig. S1 ). che-2 expression was significantly lower in C. briggsae fed on OxyS-cb-coated dead bacteria compared with that on OxyS coated (also to uncoated; Supplementary Fig. S1 ). DsrA-expressing E. coli decreases C. elegans longevity DsrA, another small ncRNA, is highly expressed in E. coli at 25 °C or below [6] , [11] ( Fig. 3a and Supplementary Fig. S3 ). We tested whether DsrA-expressing E. coli modulated C. elegans physiology by comparing the lifespan of N2 worms feeding on K12 or on DsrA deletion mutants NM6003 or DDS719. N2 worms feeding on NM6003 or DDS719 lived significantly longer than those feeding on K12 ( Fig. 3b ). These data indicated that DsrA RNA affected lifespan of C. elegans . 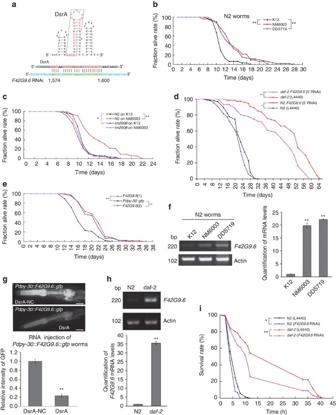Figure 3: DsrA decreases the longevity ofC. elegansby targetingF42G9.6. (a) Structure of DsrA; boxed sequence is similar toF42G9.6mRNA (up). Identical sequence in DsrA andF42G9.6mRNA (bottom); nucleotide ofF42G9.6mRNA is numbered from the start codon. (b) N2 had increased longevity on DsrA mutant strains than on thewild-typeK12. (c) Compared with N2 worms,F42G9.6(tm2908) worms had decreased longevity on K12, and showed no significant difference on longevity when fed with K12 or DsrA mutant.tm3026gave similar results astm2908, and data were not shown.N=45 inb,c. (d)F42G9.6feeding RNAi decreased longevity in both N2 anddaf-2worms, anddaf-2worms showed more significant changes toF42G9.6feeding RNAi.N=120. (e) Overexpressing ofF42G9.6with a transgene increasedC. eleganslongevity. Data were from twoPdpy-30::F42G9.6::gfplines,F42G9.6(1) andF42G9.6(2).N=95 (Pdpy-30::gfp), 86 (F42G9.6(1)) and 44 (F42G9.6(2)). (f) Semi-quantitative PCR (left) and real-time PCR (right) showed increasedF42G9.6mRNA levels in N2 worms feeding on DsrA deletion strains. (g) Representative images (up) to show that injection of the OxyS RNA decreased GFP expression inPdpy-30::F42G9.6::gfpworms. A modified DsrA containing a scrambled sequence in the region predicted to targetF42G9.6(DsrA-NC) was used as a negative control. GFP images were taken with the same parameters. Relative quantifications of GFP signals from 20 worms were shown (bottom). Scale bar is 50 μm. (h) Semi-quantitative PCR (up) and real-time PCR (bottom) to show increasedF42G9.6 mRNA levels indaf-2worms.(i)F42G9.6feeding RNAi decreased survival rates in both N2 anddaf-2worms when challenged with paraquat to generate oxidative stress, anddaf-2worms showed more significant changes toF42G9.6feeding RNAi.N=120 for each group. The log-rank test was used to calculatePvalues for longevity and survival assays.Pvalues were determined by two-tailed Student'st-test for the other data. *P<0.05; **P<0.01. All data are from three repeats. Error bars represent s.e.m. Figure 3: DsrA decreases the longevity of C. elegans by targeting F42G9.6 . ( a ) Structure of DsrA; boxed sequence is similar to F42G9.6 mRNA (up). Identical sequence in DsrA and F42G9.6 mRNA (bottom); nucleotide of F42G9.6 mRNA is numbered from the start codon. ( b ) N2 had increased longevity on DsrA mutant strains than on the wild-type K12. ( c ) Compared with N2 worms, F42G9.6 ( tm2908 ) worms had decreased longevity on K12, and showed no significant difference on longevity when fed with K12 or DsrA mutant. tm3026 gave similar results as tm2908 , and data were not shown. N =45 in b , c . ( d ) F42G9.6 feeding RNAi decreased longevity in both N2 and daf-2 worms, and daf-2 worms showed more significant changes to F42G9.6 feeding RNAi. N =120. ( e ) Overexpressing of F42G9.6 with a transgene increased C. elegans longevity. Data were from two Pdpy-30::F42G9.6::gfp lines, F42G9.6 (1) and F42G9.6 (2). N =95 ( Pdpy-30::gfp ), 86 ( F42G9.6 (1)) and 44 ( F42G9.6 (2)). ( f ) Semi-quantitative PCR (left) and real-time PCR (right) showed increased F42G9.6 mRNA levels in N2 worms feeding on DsrA deletion strains. ( g ) Representative images (up) to show that injection of the OxyS RNA decreased GFP expression in Pdpy-30::F42G9.6::gfp worms. A modified DsrA containing a scrambled sequence in the region predicted to target F42G9.6 (DsrA-NC) was used as a negative control. GFP images were taken with the same parameters. Relative quantifications of GFP signals from 20 worms were shown (bottom). Scale bar is 50 μm. ( h ) Semi-quantitative PCR (up) and real-time PCR (bottom) to show increased F42G9. 6 mRNA levels in daf-2 worms. ( i ) F42G9.6 feeding RNAi decreased survival rates in both N2 and daf-2 worms when challenged with paraquat to generate oxidative stress, and daf-2 worms showed more significant changes to F42G9.6 feeding RNAi. N =120 for each group. The log-rank test was used to calculate P values for longevity and survival assays. P values were determined by two-tailed Student's t -test for the other data. * P <0.05; ** P <0.01. All data are from three repeats. Error bars represent s.e.m. Full size image DsrA decreases C. elegans F42G9.6 mRNA level DsrA might regulate the expression of certain genes related to C. elegans longevity. Sequence analysis showed that DsrA harbours a 27-nt (23-nt identical) sequence with similarity to the C. elegans F42G9.6 mRNA, which encodes an orthologue of diacylglycerol lipase ( Fig. 3a and Supplementary Table S1 ). F42G9.6 (tm2908 and tm3026) mutant worms lived shorter than N2 animals on K12 food ( Fig. 3c ). Feeding RNAi against F42G9.6 also decreased the lifespan of C. elegans ( Fig. 3d ). By contrast, transgenic animals overexpressing F42G9.6 promoted longevity ( Fig. 3e ). These findings demonstrated that F42G9.6 was a C. elegans longevity gene. F42G9.6 mRNA levels increased in N2 animals fed with DsrA mutant bacteria NM6003 and DDS719 ( Fig. 3f ), whereas F42G9.6 mutants did not show significant change in longevity when fed with K12 or DsrA mutant bacteria ( Fig. 3c ). We found no significant difference in longevity between worms living on dead bacteria whether they expressed DsrA or not; whereas C. elegans showed a significant decrease in longevity on DsrA RNA coated compared with negative control RNA-coated dead bacteria ( Supplementary Fig. S2 ). Real-time PCR revealed a decrease in F42G9.6 level in worms fed with DsrA-coated dead bacteria ( Supplementary Fig. S2 ). Furthermore, injection of DsrA into a Pdpy-30::F42G9.6::gfp transgenic line reduced the GFP signal ( Fig. 3g ), indicating that DsrA targeted F42G9.6 mRNA. No change in GFP levels was observed after injection of DsrA into the PF42G9.6::gfp transgenic line. Therefore, DsrA inhibits F42G9.6 posttranscriptionally to reduce the longevity of C. elegans . Requirement of the genuine F42G9.6 promoter in this suppression is excluded with a foreign promoter in the Pdpy-30::F42G9.6::gfp reporter line, but we could not rule out the possibility of inhibition at the transcriptional level requiring the genomic coding region or the nascent transcript of F42G9.6 . F42G9.6 phenotype is related to the daf-2 pathway daf-2 , a hormone receptor in C. elegans similar to the insulin and IGF-1 receptors, influences lifespan of the animal by regulating gene expression [12] . F42G9.6 expression was upregulated in the daf-2 mutant ( Fig. 3h ). On the other hand, F42G9.6 knockdown with RNAi partially blocked daf-2 longevity and oxidative stress resistance when paraquat was used to generate oxidative stress in the oxidative stress resistance assays [13] ( Fig. 3d ). Thus, F42G9.6 is probably a longevity gene in the daf-2 pathway. Several other C. elegans genes, such as pgp-5 , sma-1 , srd-71, srd-72 , C14C10.5 and fax-1 , have sequences complementary to DsrA or a similar sequence in their mRNA coding region. pgp-5 , but not sma-1 or fax-1 , may also be regulated by DsrA, as pgp-5 mRNA levels were increased in N2 worms fed with DsrA mutant bacteria ( Supplementary Fig. S4 ). OxyS and DsrA show a distinct requirement for RNAi genes We compared the repelling effect of OxyS in wild-type worms with that in mutants of the RNAi pathway [5] using food comparison assays. We examined nine RNAi genes these included: dcr-1 that encodes a bidentate ribonuclease with homologues in essentially all animals and cuts dsRNAs into small interference RNAs or microRNA precursor into mature microRNA [5] . alg-1 and alg-2 are argonaute genes involved in microRNA pathway [5] . rde-1 is an argonaute gene involved in the feeding RNAi pathway [5] . rde-2 is a gene specific for Caenorhabditis involved in RNAi and transposon silencing [5] . rde-4 encodes a Caenorhabditis -specific dsRNA-binding protein, and functions during the initiation phase of RNAi [5] . rrf-3 is an RNA-dependent RNA polymerase gene specific for Caenorhabditis , and a negative regulator for feeding RNAi [5] . sid-1 encodes a dsRNA channel with human and mouse homologues [5] , [14] . sid-2 is a C. elegans -specific single-pass transmembrane protein gene required for dsRNA-based feeding RNAi [5] , [15] . On the basis of the observed repelling effect of OxyS in these mutants, it appeared that alg-1 and rde-4 had major roles in this repulsion; dcr-1 , rde-1 and rde-2 had some effects; alg-2 , sid-1 and sid-2 might be irrelevant or redundant ( Fig. 4a ). che-2 mRNA levels in alg-1 and rde-4 mutants fed continuously with OxyR E. coli did not change significantly compared with mutant worms fed with K12 ( Fig. 4b ), whereas alg-2 , rrf-3 , sid-1 and sid-2 mutants still showed significant changes in che-2 mRNA levels as compared with N2 ( Fig. 4c ). Thus, we proposed that OxyS might utilize a pathway requiring alg-1 and rde-4 . We also investigated the involvement of ABC transporters, haf-2 and haf-6 [16] . Data indicated that haf-2 but not haf-6 was required for the effect of OxyS in C. elegans ( Fig. 4d ). The repelling effect of OxyS did not increase in RNAi enhancer mutants including rrf-3(pk1426) , eri-1(mg366) , eri-3(tm1361) and eri-9(gg106 ; data not shown). Notably, in food searching ability and food comparison assays, the effect of OxyS-expressing E. coli on C. elegans was more prominent than that of bacteria expressing che-2 dsRNA ( Fig. 4f ). This finding was further confirmed by assessing che-2 mRNA levels by real-time PCR ( Fig. 4h ). Injection of the 17-nt-complementary single-stranded small RNA (ssRNA) into Pche-2::che-2::gfp worms also reduced the GFP signal ( Fig. 4i ), although to a lesser degree than the decrease by the injection of full length OxyS or the feeding of OxyS-expressing E. coli . We also injected 17nt small RNAs targeting to C. briggsae che-2 ( cb-che-2 ), and found these small RNAs could downregulate cb-che-2 ( Supplementary Fig. S1 ). We confirmed the speculation that the effect of dsRNA feeding RNAi against che-2 was irrelevant with alg-1 and alg-2 , and dependent on dcr-1 , rde-1 , rde-2 , rde-4 , sid-1 and sid-2 ( Supplementary Fig. S5 ). rrf-3 was a negative regulator for the effect of dsRNA feeding RNAi against che-2 ( Supplementary Fig. S5 ). These results are consistent with known roles of these genes in the feeding RNAi pathway [5] . 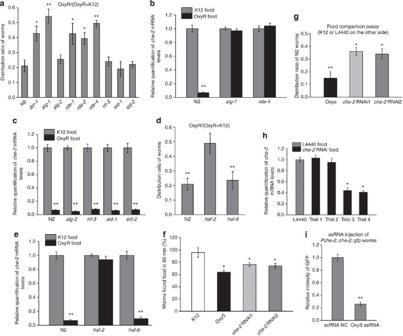Figure 4: Involvement of RNAi genes in the effects of OxyS onC. elegans. (a) Repelling effect of OxyRE. colion various mutants of theC. elegansRNAi/microRNA pathways in food comparison assays.N=36 worms for each group. (b)che-2mRNA levels in N2,alg-1andrde-4worms were shown by real-time PCR. (c) Levels ofche-2mRNA inalg-2,rrf-3,sid-1andsid-2worms fed with K12 and OxyR food. Inaandc, two alleles ofsid-1 (qt2&pk3321) andsid-2(qt42&gk505) were examined, and data from only one allele for each gene (pk3321andqt42) were presented, as both alleles of each gene gave similar results. (d)haf-6but nothaf-2mutant showed similar distribution as N2 worms in the food comparison assays.N=36 worms. (e) OxyS had no effect on the level ofche-2mRNA inhaf-2worms, whereas the suppressive effect was present inhaf-6worms. (f) Comparison of food searching ability for worms fed on OxyS orche-2RNAi bacteria.N=40 worms for each group. (g) Worms fed on OxyS orche-2RNAi bacteria examined with food comparison assay.N=36 worms for each group. (h) Real-time PCR ofche-2mRNA levels to compare the effect of OxyS toche-2dsRNA-based feeding RNAi. Ine–h, 2 out of 10 trials withche-2feeding RNAi showed significant effect in behavioural tests, and the data shown were from these two trials only. (i) Injection of the 17-nt complementary ssRNA suppressed the expression ofPche-2::che-2::gfp. Scramble small RNA (scRNA NC) was used as a negative control.N=20 worms for each group.Pvalues were determined by two-tailed Student'st-test. *P<0.05; **P<0.01. All data are from three repeat experiments. Error bars represent s.e.m. Figure 4: Involvement of RNAi genes in the effects of OxyS on C. elegans . ( a ) Repelling effect of OxyR E. coli on various mutants of the C. elegans RNAi/microRNA pathways in food comparison assays. N =36 worms for each group. ( b ) che-2 mRNA levels in N2, alg-1 and rde-4 worms were shown by real-time PCR. ( c ) Levels of che-2 mRNA in alg-2 , rrf-3 , sid-1 and sid-2 worms fed with K12 and OxyR food. In a and c , two alleles of sid -1 ( qt2 & pk3321 ) and sid-2 ( qt42 & gk505 ) were examined, and data from only one allele for each gene ( pk3321 and qt42 ) were presented, as both alleles of each gene gave similar results. ( d ) haf-6 but not haf-2 mutant showed similar distribution as N2 worms in the food comparison assays. N =36 worms. ( e ) OxyS had no effect on the level of che-2 mRNA in haf-2 worms, whereas the suppressive effect was present in haf-6 worms. ( f ) Comparison of food searching ability for worms fed on OxyS or che-2 RNAi bacteria. N =40 worms for each group. ( g ) Worms fed on OxyS or che-2 RNAi bacteria examined with food comparison assay. N =36 worms for each group. ( h ) Real-time PCR of che-2 mRNA levels to compare the effect of OxyS to che-2 dsRNA-based feeding RNAi. In e – h , 2 out of 10 trials with che-2 feeding RNAi showed significant effect in behavioural tests, and the data shown were from these two trials only. ( i ) Injection of the 17-nt complementary ssRNA suppressed the expression of Pche-2::che-2::gfp . Scramble small RNA (scRNA NC) was used as a negative control. N =20 worms for each group. P values were determined by two-tailed Student's t -test. * P <0.05; ** P <0.01. All data are from three repeat experiments. Error bars represent s.e.m. Full size image We examined the longevity-decreasing effect of DsrA in mutants of the RNAi pathway [5] . rde-4 was required for the effect of DsrA as the longevity-decreasing effect of DsrA in rde-4 ( ne301 ) worms was not as prominent as in N2 worms ( Fig. 5a ). Other genes, including sid-1 and sid-2 , might be irrelevant or redundant to the DsrA effect as mutant worms were sensitive to the longevity-decreasing effect of K12 E. coli (data not shown). The effect of rde-2 is rather intriguing in that rde-2 mutants lived moderately longer on K12, but showed a much greater increase in longevity on NM6003 food than N2 worms ( Fig. 5b ). The rde-4 mutant showed a smaller increase, whereas rde-2 mutant showed a much greater increase in the F42G9.6 mRNA level on NM6003 food ( Fig. 5c ). We performed real-time PCR and found alg-2 , rrf-3 , sid-1 and sid-2 mutant were similar to N2 for the effect of DsrA on F42G9.6 . ( Fig. 5d ). The data also indicated that ABC transporter haf-6 but not haf-2 was required for the effect of DsrA in C. elegans ( Fig. 5e ). We also confirmed that the effect of dsRNA feeding RNAi against F42G9.6 was independent of alg-1 and alg-2 , and dependent on dcr-1 , rde-1 , rde-2 , rde-4 , sid-1 and sid-2 ( Supplementary Fig. S5 ). rrf-3 was a negative regulator for the effect of dsRNA feeding RNAi against F42G9.6 ( Supplementary Fig. S5 ). 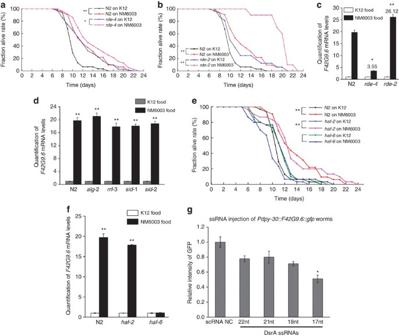Figure 5: Involvement of RNAi genes in the effects of DsrA onC. elegans. (a)rde-4 (ne301)worms did not show marked changes in longevity when fed with K12 or DsrA mutant (NM6003)E. colicomparing with N2 worms, suggesting thatrde-4is involved in the effect of DsrA RNA inC. elegans. (b)rde-2(pk1657)worms showed an increase lifespan compared with N2 when fed with DsrA mutant (NM6003) versus K12E. coli.N=45 worms for each group ina,b. (c) Real-time PCR results revealed thatrde-4mutant showed a lower increase inF42G9.6mRNA level, whereasrde-2mutant showed much greater increase inF42G9.6mRNA level on NM6003 food. The actual values ofF42G9.6forrde-4andrde-2on NM6003 food were labelled. (d) Levels ofF42G9.6mRNA inalg-2,rrf-3,sid-1andsid-2worms fed with K12 and NM6003 (DsrA deletion strain) food. (e) ABC transporterhaf-2but nothaf-6mutant showed a similar longevity effect as N2 worms.N=60 worms for each group. (f) Real-time PCR revealed that DsrA had no effect on the level ofF42G9.6mRNA inhaf-6worms, whereas the increase on the level ofF42G9.6mRNA was seen inhaf-2and N2 worms when fed with DsrA mutant NM6003. (g) Injection of the 17-22-nt complementary ssRNAs (DsrA ssRNAs) intoPdpy-30::F42G9.6::gfpworms. The 17-nt ssRNA suppressed the expression ofPche-2::che-2::gfp. Scramble small RNA (scRNA NC) was used as a negative control. GFP images were taken with same parameters.N=20 worms for each group. The log-rank test was used to calculatePvalues for longevity assays. The Student'st-test was used to calculate thePvalues for other data. *Pvalue <0.05; **Pvalue <0.01. All data are from three repeat experiments. Error bars represent s.e.m. Figure 5: Involvement of RNAi genes in the effects of DsrA on C. elegans . ( a ) rde-4 (ne301) worms did not show marked changes in longevity when fed with K12 or DsrA mutant (NM6003) E. coli comparing with N2 worms, suggesting that rde-4 is involved in the effect of DsrA RNA in C. elegans . ( b ) rde-2(pk1657) worms showed an increase lifespan compared with N2 when fed with DsrA mutant (NM6003) versus K12 E. coli . N =45 worms for each group in a , b . ( c ) Real-time PCR results revealed that rde-4 mutant showed a lower increase in F42G9.6 mRNA level, whereas rde-2 mutant showed much greater increase in F42G9.6 mRNA level on NM6003 food. The actual values of F42G9.6 for rde-4 and rde-2 on NM6003 food were labelled. ( d ) Levels of F42G9.6 mRNA in alg-2 , rrf-3 , sid-1 and sid-2 worms fed with K12 and NM6003 (DsrA deletion strain) food. ( e ) ABC transporter haf-2 but not haf-6 mutant showed a similar longevity effect as N2 worms. N =60 worms for each group. ( f ) Real-time PCR revealed that DsrA had no effect on the level of F42G9.6 mRNA in haf-6 worms, whereas the increase on the level of F42G9.6 mRNA was seen in haf-2 and N2 worms when fed with DsrA mutant NM6003. ( g ) Injection of the 17-22-nt complementary ssRNAs (DsrA ssRNAs) into Pdpy-30::F42G9.6::gfp worms. The 17-nt ssRNA suppressed the expression of Pche-2::che-2::gfp . Scramble small RNA (scRNA NC) was used as a negative control. GFP images were taken with same parameters. N =20 worms for each group. The log-rank test was used to calculate P values for longevity assays. The Student's t -test was used to calculate the P values for other data. * P value <0.05; ** P value <0.01. All data are from three repeat experiments. Error bars represent s.e.m. Full size image As DsrA harbours a sequence with similarity to F42G9.6 mRNA, one would expect that antisense RNA complementary to F42G9.6 mRNA must exist to mediate the inhibition of DsrA on F42G9.6 . Analysis of published deep sequencing data showed that small RNAs corresponding to both DsrA sense and antisense sequences were present in C. elegans [17] ( Supplementary Table S2 ). Actually, deep sequencing revealed more small RNAs corresponding to DsrA antisense than sense sequence, with a ratio of antisense: sense of ~4:1 in L1 worms, 4:1 in L2 worms and 2:1 in L3 worms ( Supplementary Table S2 ). The mechanism for the generation of DsrA antisense RNAs in C. elegans remains to be clarified. We injected four individual ssRNAs with length from 17 to 22nt complementary to F42G9.6 mRNA into C. elegans , and found the 17-nt RNA reduced GFP signals of Pdpy-30::F42G9.6::gfp transgenic line ( Fig. 5g ). OxyS and DsrA have protective effects to E. coli We examined the possible protective effects of OxyS and DsrA on E. coli under the foraging pressure of C. elegans . When equal numbers of K12 and OxyS bacteria was seeded onto the same plate ( Fig. 6a ), more OxyS bacteria than K12 were left over a period of 5 days under the foraging of C. elegans , even though OxyS strain grows slower than K12 on the no-worm control plates ( Fig. 6a ). We also fed C. elegans an equal number of K12 and NM6003 DsrA deletion bacteria on separate plates, and examined the mutual impact between C. elegans and bacteria ( Fig. 6b ). After 2 weeks, there were fewer worms on K12 than on NM6003 plates ( Fig. 6b ), and there were more bacteria in K12 than NM6003 plates ( Fig. 6c ). In the no-worm control, DsrA mutants grow slower than K12, but the ratios of K12 to NM6003 on the plates with worms were significantly higher than those on no-worm control plates ( Fig. 6c ). These results indicated a protective role of OxyS and DsrA to E. coli under the foraging of C. elegans . 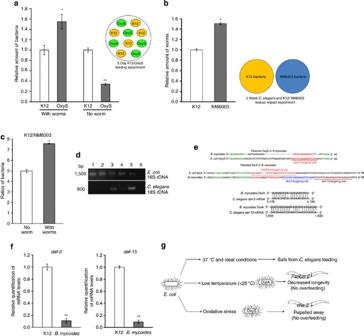Figure 6: Mutual impact betweenC. elegansandE. coliand a model of the relationship mediated by ncRNAs betweenE. coliandC. elegans. (a) Relatively more OxyS bacteria than K12 were left over a period of 5 days under the forage ofC. elegans, even though OxyS grew slower than K12 bacteria on no-worm plates. Setup for the 5-day feeding experiment is shown at right. (b) Fewer worms on K12 than on NM6003 bacteria after a feeding period of 2 weeks. Setup for the experiment is shown at right. (c) The ratios of K12 to NM6003 bacteria onC. elegansforage plates were significantly higher than those ratios on no-worm control plates after a period of 2 weeks. (d) PCR of species-specific rDNA sequences showed coexistence ofC. elegansandE. coliin three samples from the wild. There wasE. colibut noC. elegansdetected for samples 1 and 2;E. coliandC. eleganswere co-detected in samples 3, 4 and 5; lane 6 was no-template control. (e) PotentialB. mycoidesOxyS sequence aligned withE. colihomologue, andC. elegans che-2-targeting site inE. coliOxyS is underlined (top). DsrA sequences fromE. coliandB. mycoidesare shown (middle), with labelling ofF42G9.6-targeting site (dotted line),daf-2-targeting site (dashed line) anddaf-15-targeting site (solid line). Alignments betweenB. mycoidesDsrA andC. elegans daf-2/daf-15mRNA are also shown (bottom). (f) Levels ofdaf-2(left) anddaf-15mRNA (right) inC. elegansfeeding onB. mycoideswere lower than those on K12E. coli. (g) A model ofE. coli/C. elegansinteraction mediated byE. colincRNAs. The Student'st-test was used to calculate thePvalues. *Pvalue <0.05; **Pvalue <0.01. All data are from three repeat experiments. Error bars represent s.e.m. Figure 6: Mutual impact between C. elegans and E. coli and a model of the relationship mediated by ncRNAs between E. coli and C. elegans . ( a ) Relatively more OxyS bacteria than K12 were left over a period of 5 days under the forage of C. elegans , even though OxyS grew slower than K12 bacteria on no-worm plates. Setup for the 5-day feeding experiment is shown at right. ( b ) Fewer worms on K12 than on NM6003 bacteria after a feeding period of 2 weeks. Setup for the experiment is shown at right. ( c ) The ratios of K12 to NM6003 bacteria on C. elegans forage plates were significantly higher than those ratios on no-worm control plates after a period of 2 weeks. ( d ) PCR of species-specific rDNA sequences showed coexistence of C. elegans and E. coli in three samples from the wild. There was E. coli but no C. elegans detected for samples 1 and 2; E. coli and C. elegans were co-detected in samples 3, 4 and 5; lane 6 was no-template control. ( e ) Potential B. mycoides OxyS sequence aligned with E. coli homologue, and C. elegans che-2 -targeting site in E. coli OxyS is underlined (top). DsrA sequences from E. coli and B. mycoides are shown (middle), with labelling of F42G9.6 -targeting site (dotted line), daf-2 -targeting site (dashed line) and daf-15 -targeting site (solid line). Alignments between B. mycoides DsrA and C. elegans daf-2 / daf-15 mRNA are also shown (bottom). ( f ) Levels of daf-2 (left) and daf-15 mRNA (right) in C. elegans feeding on B. mycoides were lower than those on K12 E. coli . ( g ) A model of E. coli / C. elegans interaction mediated by E. coli ncRNAs. The Student's t -test was used to calculate the P values. * P value <0.05; ** P value <0.01. All data are from three repeat experiments. Error bars represent s.e.m. Full size image ncRNA-mediated bacteria/bacteria forager interaction Although C. elegans is generally raised on E. coli in laboratories, these bacteria are not considered as a major C. elegans food source in nature [18] . We isolated wild C. elegans in three rotten plant samples; in all these three cases, E. coli was also detected ( Fig. 4d ). In addition, in a confined laboratory space, mice could spread C. elegans and E. coli ( Supplementary Fig. S6 ). Sequences similar to OxyS and DsrA were identified in soil bacteria Bacillus ( Fig. 4e ), which may presumably make up part of the major food sources for C. elegans in the wild [19] . OxyS similar sequences in Bacillus mycoides (Bm-OxyS) contain a 15-nt ' che-2 -targeting' site ( Fig. 6e ). We doubt this 15nt site is sufficient to suppress C. elegans che-2 as che-2 mRNA level of worms on B. mycoides is similar to that on ΔOxyS E. coli , and both are much higher than that of worms on OxyS E. coli (not shown). The similar sequences in B. mycoides (Bm-DsrA) do not contain the ' F42G9.6 -targeting' site; instead, the sequences harbour a 21-nt site complementary to C. elegans daf-2 mRNA and a 25-nt site complementary to C. elegans daf-15 mRNA ( Fig. 6e ). Whether Bm-DsrA is expressed as small ncRNAs or it executes anti-oxidative functions in B. mycoides remains to be determined. B. mycoides may be a preferred bacterial species to C. elegans [20] , [21] , and lifespan of C. elegans is longer on B. mycoides than on E. coli [21] , indicating a possibility that Bm-DsrA suppresses the expression of daf-2 and/or daf-15 in C. elegans , as loss-of-function mutants of daf-2 or daf-15 extend C. elegans longevity [12] . Indeed, worms fed on B. mycoides had lower daf-2 and daf-15 mRNA levels than on E. coli ( Fig. 6f ). Whether Bm-DsrA has roles in the possible mutual impact between B. mycoides and C. elegans remains to be investigated. Both OxyS and DsrA are expressed in E. coli under stress conditions, and we propose a model where these bacterial ncRNAs may have interspecies functions in ecosystem. E. coli could 'utilize' these ncRNAs as a means to protect themselves under harsh environments from overforaging by C. elegans ( Fig. 6g ). By identifying two endogenous E. coli ncRNAs OxyS and DsrA and demonstrating their physiological effects on C. elegans via regulating gene expression, we have described a potential new mode of RNA-mediated bacteria/bacteria forager interaction. It seems that both OxyS and DsrA require rde-4 , a dsRNA-binding protein gene, while they showed distinct dependence on other known RNAi genes in C. elegans . ABC transporters, haf-2 and haf-6 , are required, respectively, for the effect of OxyS and DsrA in C. elegans ( Figs 4d and 5e,f ). The reason for this difference is unknown. Different expression patterns of haf-2 and haf-6 might mediate their functional distinctions [16] . We could not definitively rule out the involvement of other known RNAi-related genes and pathways due to the nature of alleles we used and potential redundancy among these genes. It seems that a 17-nt antisense small RNA is sufficient to suppress the expression of che-2 or F42G9.6 ( Figs 4i and 5g ), although it is also possible that the gene suppression by injected 17nt ssRNAs could be an antisense effect. However, we need to be cautions when interpreting the effect observed after injection due to technical features (acute effect from high concentration of injected RNA or injury from injection). The roles of sid-1 and sid-2 in C. elegans feeding RNAi with bacteria harbouring engineered dsRNA are well established [3] , [14] , [15] . It was a surprise to us that our data indicated that sid-1 and sid-2 are not necessary (or maybe redundant) for the effects of OxyS and DsrA on C. elegans . ABC transporters are found to transport a wide variety of substrates such as sugars, amino acids, metal ions, peptides and proteins [22] . We do not know the exact molecular mechanism for the role of ABC transporters in the effect of OxyS and DsrA on C. elegans . It is interesting that rde-4 was recently found to be essential for transgenerational inheritance of small RNA-based antiviral response in C. elegans [23] . There are endogenous 17-18nt small ncRNAs originating from transcription initiation and splice sites in metazoans including C. elegans [24] , although functional study of this kind of ncRNAs has not been investigated. In Drosophila zygotic transition, piRNA could downregulate maternal mRNAs by 16 bp complementary between piRNAs and 3′UTR of maternal mRNA (continuous 16 bp complementary or 5+11 bp complementary disrupted by 1 bp of mismatch) [19] . Short interfering RNAs originating from viruses were recently found to have roles in the interactions between viruses and plant cells [25] , [26] . Efforts are needed for further characterization of the molecular mechanisms behind the effects of OxyS and DsrA on C. elegans . Our data indicated the possible co-existence of E. coli and C. elegans in ecosystems ( Fig. 6d ). Invertebrates [27] and other animals (for example, mice, Supplementary Fig. S6 ) could potentially carry C. elegans around, and at the same time spread E. coli into their ecosystems [28] . Although E. coli may not be a major natural food of C. elegans , they could have encountered each other for millions of years, and the interaction between them could be one of the multiple driving forces behind the evolution of both species. C. elegans may be an opportunistic forager in the wild, accepting any bacteria including E. coli that have no acute killing effect. The interspecies effects of OxyS and DsrA, secondary to its primary regulatory roles in bacterial stress responses, may have been formed during the course of co-evolution between bacteria (for example, E. coli and B. mycoides ) and bacteria forager (for example, C. elegans ). The relevant ' C. elegans -targeting sequences' in both OxyS and DsrA are distinct from the ' E. coli functional segments' of these RNAs ( Figs 2a and 4a ), indicating the ' C. elegans -targeting' effects of these RNAs are probably secondary adaptations. Although our data showed a role of E. coli ncRNAs on C. elegans , we could not exclude that 'stressed out' bacteria also produced toxic metabolites to affect C. elegans at the same time. Our research indicates that bacteria could utilize their ncRNAs for an interspecies ecologic role to affect bacteria foragers for the possible benefit of bacteria ( Fig. 6 ). Recently, a report indicated that plant microRNAs in the food of animals could have interspecies roles in mammalian cells [29] . Exogenous dsRNA-based feeding RNAi has been used in bacteria and plants as a biotechnology against nematodes and insects [30] , [31] . Our work provides a paradigm of interspecies gene regulation and physiological modulation initiated by endogenous ncRNAs in E. coli against C. elegans . Culture of worms For routine purpose, animals were grown at 20 °C on nematode growth medium (NGM), provided with OP50 as their food unless specified. The strains used were as follws: wild-type Bristol strain N2, dcr-1(mg375), che-2(e1033), alg-1(gk214), alg-2(ok304), rde-1(ne219), rde-2(pk1657), rde-4(ne301), rrf-3(pk1426) , eri-1(mg366) , eri-3(tm1361) , sid-1 ( qt2 and pk3321 ), sid-2 ( qt42 and gk505) , eri-9(gg106) , daf-2(e1370) , F42G9.6 mutants ( tm2908 and tm3026 ), haf-2(gk13) , haf-6(ok3219) , Pche-2::che-2::gfp;rol-6 transgenic line [10] , Pche-2::gfp transgenic lines, Pdpy-30::F42G9.6::gfp transgenic lines, Pdpy-30::gfp transgenic lines, PF42G9.6::gfp transgenic lines and C. briggsae . Bacterial strains OP50, used for general culture of worms. HT115 (with L4440 feeding RNAi vector or gene-specific dsRNA plasmid), used for dsRNA-based feeding RNAi. K12, wild-type E. coli , used as a control for most experiments. oxyR2 (named as OxyR in the text), a constitutive oxyR2 mutant, expressing oxyS constitutively [8] . JM109/PKK177.3-oxyS (named as OxyS in the text), a strain overexpressing OxyS due to a recombinant OxyS plasmid it harbors [8] . MC4100/oxyS − (named as ΔOxyS in the text), OxyS deletion strain [8] . NM6003 and DDS719 are DsrA deletion mutants. The genotype of NM6003 is F-, [araD139] B/r , Δ(argF-lac)169 , &lambda − , ΔdsrA5 , zed-3069::Tn10 , rph-1 ; DDS719 is F-, [araD139] B/r , Δ(argF-lac)169 , &lambda − , LAMdsrB::lacZ(DDS314) , e14 -, flhD5301 , ΔdsrA5 , zed-3069::Tn10 , Δ(fruK-yeiR)725(fruA25) , relA1 , rpsL150 (strR), rbsR22 , Δ(fimB-fimE)632(::IS1) , deoC1 . B. mycoides was also used as food for C. elegans in some experiments. C. elegans behavioural assays In food quality assay, N2 worms were raised on OP50 bacteria. The experimental 60-mm NGM plates were prepared the day before, with the corresponding food (K12, OxyR, OxyS or ΔOxyS) dropped at one end of the plates. Tested worms were picked and transferred to clean NGM plates for the deprivation of food for 30 min. Then worms were placed at the end opposite to the bacteria, and worms staying on each food spot were quantified and recorded at 60 min. In food comparison assay, N2 worms were raised on OP50 bacteria. The experimental 60-mm NGM plates were prepared with K12 and one of the other strains (OxyS, OxyR or ΔOxyS) at two opposite ends of the plates the day before. Tested worms were transferred to clean plates and deprived of food for 30 min. Then the same number of worms was placed on food at each end of the testing plates, and worms staying on each food were quantified and recorded at 2, 12, 24 and 36 h, respectively. In food comparison assays, che-2 null mutant could not stay on both sides of the food, and generally >90% of worms in the assays run off from food and ended up dead (or disappeared) within 12 h (data not shown). Therefore, mutants such as che-2 null allele with serious chemosensory defects could not be subjected to food comparison assays. Thus, all mutants we showed data with could complete the food comparison assays, indicating that these mutants had at least chemosensory ability to stay on food (not wondering off and get lost) if there was no factors such as OxyS to compromise their chemosensory ability. In food searching ability assay, N2 worms were raised on K12, OxyS or OxyR bacteria for 2 days, respectively. The experimental 60-mm NGM plates were prepared the day before, with OP50 bacteria dropped at one end of the plates. Tested worms were picked, transferred to clean NGM plates and deprived of food for 30 min. Then worms were placed at the end opposite to the bacteria, and worms staying on each food spot were quantified and recorded at 90 min. In chemo-attractive assay with NaCl, N2 worms were raised on K12, OxyS or OxyR bacteria for 2 days, respectively. The experimental 60-mm NGM plates were prepared before use, with NaCl gradients dropped at one end of the plates. Tested worms were picked, transferred to clean NGM plates and deprived of food for 30 min. Then worms were placed at the end opposite to NaCl gradients, and worms staying on NaCl were quantified and recorded at 90 min. In chemo-avoidance assay with copper acetate, N2 worms were raised on K12, OxyS or OxyR bacteria for 2 days, respectively. The experimental 60-mm NGM plates were prepared before use, with copper acetate barrier in the middle of the plates. Tested worms were picked, transferred to clean NGM plates and deprived of food for 30 min. Then worms were placed at one end opposite to copper acetate barrier, and worms staying on copper acetate were quantified and recorded at 90 min. Experiments with dead bacteria E. coli bacteria were killed with boiling or UV treatment [32] . For food comparison assay, two dead bacterial spots were placed on opposite sides of the plate. In assays with dead bacteria coated with in vitro synthesized RNA, we added 10 μl RNA (concentration 5 μg μl −1 , with RNase inhibitor) onto the food spot. Fresh RNA was added every day for longevity assays. Long-term OxyS protective effect experiment Equal amounts of K12 and OxyS E. coli , each five drops, were put on the same 60-mm NGM plates overnight. Four L4 hermaphrodites were transferred onto the plate, and these worms along with their progeny fed on the plate for 5 days. No-worm control plates were also set up with equal amount of K12 and OxyS E. coli on NGM plates for 5 days. Plates were washed with phosphate-buffered saline, and the amount of bacteria was calculated based on bacteria clones from serial dilutions. K12 and OxyS (ampR) E. coli can be distinguished from each other based on the amp R of OxyS E. coli . Data were collected from three repeats. Long-term mutual impact between worm and E. coli strains Equal amount of K12 and NM6003 E. coli was spread on separate 150-mm NGM plates. Two L4 hermaphrodites were transferred onto the plate the next day, and these worms along with their progeny fed on the plate for 2 weeks. No-worm control plates were also set up with equal amount of K12 and NM6003 on NGM plates for 2 weeks. Worms on each plate were then counted. Plates were then washed with phosphate-buffered saline, and the amount of bacteria was calculated based on bacteria clones from serial dilutions. Data were collected from three repeats. Coexistence of C. elegans and E. coli in nature Rotten plant samples (fruits and nutritional roots) from orchards and rural forests around Wuhan and Hefei (two cities in central China) were collected with caution to avoid contamination. For collecting rotten plant samples, we worn plastic one-time-use sterilized gloves and used sterilized plastic bags to keep individual samples from contamination from hands and environment, and from contamination among samples. A portion of individual samples was cut out and put on a 10-cm NGM plate seeded with OP50. Plates were checked for the presence of worms 4 days later. Four individual worms appearing to be C. elegans were picked out from each plate and were used as template for PCR reaction without the extraction of genomic DNA with a pair of primers specific for the C. elegans 18S rDNA with an amplicon size of 0.8 kb. We then performed PCR with remaining portion of samples collected (kept under −86 °C) using a pair of primers specific for the E. coli 16S rDNA with a 1.5-kb amplicon. In vitro synthesis of RNA To generate appropriate template for in vitro transcription, a PCR product was amplified from OxyS or OxyS-cb plasmid or E. coli genomic DNA (for DsrA) with the corresponding primer pairs, which contained T7 promoter. OxyS, OxyS-cb and DsrA RNA were made by in vitro transcription with T7 RNA polymerase using the above PCR products as template. OxyS-NC and DsrA-NC were synthesized with the same method except that the site predicted to target che-2 and F42G9.6 was changed to a scramble sequence. Primers used for in vitro synthesis of RNA and other molecular assays are listed in the Supplementary Table S3 . RNA injection into worms RNA was injected into intestinal cavity of worms. OxyS and DsrA RNA was injected at 1 μg μl −1 into Pche-2::che-2::gfp ; rol-6 and Pdpy-30::F42G9.6::gfp C. elegans at the L4 stage, respectively. OxyS-NC and DsrA-NC modified at the site predicted to target che-2 and F42G9.6 , respectively, into a scramble sequence were used as negative controls. The 17-nt (5′-CGUUUCGAGAGUUUCUC-3′) RNA oligo complementary to che-2 mRNA, 17nt (5′-CAAGAAGCACUUAAAAA-3′), 18nt (5′-CAAGAAGCACUUAAAAAA-3′), 21nt (5′-AAGAAGCACUUAAAAAAUUCG-3′) and 22nt (5′-CAAGAAGCACUUAAAAAAU UCG-3′) RNA oligo complementary to F42G9.6 mRNA were injected at concentration of 1.2 μg μl −1 into Pche-2::che-2::gfp ; rol-6 and Pdpy-30::F42G9.6::gfp worms at the L4 stage, respectively, and scramble RNA oligo was used as a negative control for injection. Worms were recovered from injection for 30 h and then subjected to imaging. The 17-nt (5′-CGUUUCGAGAGUUUCUC-3′) RNA oligo complementary to cb-che-2 mRNA was injected into C. briggsae at 1 μg μl −1 , and the 17-nt RNA oligo complementary to C. elegans che-2 mRNA was used for comparison. C. briggsae were recovered from injection for 30 h and then subjected to RNA isolation and real-time PCR to examine the cb-che-2 expression level. How to cite this article: Liu, H. et al . Escherichia coli noncoding RNAs can affect gene expression and physiology of Caenorhabditis elegans . Nat. Commun. 3:1073 doi: 10.1038/ncomms2071 (2012).